PCAF-dependent epigenetic changes promote axonal regeneration in the central nervous system Axonal regenerative failure is a major cause of neurological impairment following central nervous system (CNS) but not peripheral nervous system (PNS) injury. Notably, PNS injury triggers a coordinated regenerative gene expression programme. However, the molecular link between retrograde signalling and the regulation of this gene expression programme that leads to the differential regenerative capacity remains elusive. Here we show through systematic epigenetic studies that the histone acetyltransferase p300/CBP-associated factor (PCAF) promotes acetylation of histone 3 Lys 9 at the promoters of established key regeneration-associated genes following a peripheral but not a central axonal injury. Furthermore, we find that extracellular signal-regulated kinase (ERK)-mediated retrograde signalling is required for PCAF-dependent regenerative gene reprogramming. Finally, PCAF is necessary for conditioning-dependent axonal regeneration and also singularly promotes regeneration after spinal cord injury. Thus, we find a specific epigenetic mechanism that regulates axonal regeneration of CNS axons, suggesting novel targets for clinical application. The regenerative response initiated following axonal injury in the peripheral nervous system (PNS) versus the central nervous system (CNS) leads to differential growth capacities and repair. In fact, the lack of pro-neuroneal growth gene expression and glial inhibitory signals leads to regenerative failure following CNS but not PNS injury [1] , [2] , [3] , [4] . Immediately after a peripheral nerve injury, rapid ion fluxes increase, followed by a rise in cAMP levels, axonal translation occurs, phosphorylation retrograde cascades activate transcription factors, gene expression is induced and finally regeneration occurs [5] , [6] . However, the final link between axonal injury-induced retrograde signalling and the regulation of essential regenerative gene expression remains elusive. The dorsal root ganglia (DRG) sensory neurone system has a central as well as a peripheral axonal branch departing from a single cell body. This allows for bimodal injury inputs with differing regenerative capacities into one central transcriptional hub. Interestingly, the lack of regeneration of injured ascending sensory fibres in the spinal cord can be partially enhanced by an injury to the peripheral branch (conditioning lesion) of DRG neurones [7] . In search of key regulatory mechanisms that may clarify the molecular nature of this regenerative gene expression programme, we hypothesized that as an ‘orchestrator of gene regulation’ epigenetic changes would direct expression of genes crucial for regeneration only in the presence of pro-regenerative signalling following peripheral but not central damage. Identification of a specific regulatory mechanism shared by several essential genes may lead to novel molecular strategies recapitulating the conditioning effect, thus non-surgically enhancing axonal regeneration in the CNS. To this end, we employed the first systematic approach to understand the epigenetic environment in DRG neurones. We examined both DNA methylation and various key histone modifications with regards to gene regulation following axonal injury. We found that p300/CBP-associated factor (PCAF)-dependent acetylation of histone 3 lysine 9 (H3K9ac), paralleled by a reduction in methylation of H3K9 (H3K9me2), occurred at the promoters of select genes only after PNS axonal injury. In addition, we observed that extracellular signal-regulated kinase (ERK) axonal retrograde signalling is required for PCAF-dependent acetylation at these promoters and for their enhancement in gene expression. Finally, we established that PCAF is required for regeneration following a conditioning lesion and PCAF overexpression promotes axonal regeneration similar to that of a conditioning lesion after CNS injury in spinal ascending sensory fibres. Our results show the first evidence of immediate retrograde signalling leading to long-term epigenetic reprogramming of gene expression of select genes whose modulation leads to axonal regeneration in the hostile spinal environment. Histone codes are shaped by a peripheral not by a central lesion Given that epigenetic changes are a rapid and dynamic way to translate external stimuli into targeted and long-lasting gene regulation, such has been observed in learning and memory, seizures, stroke and neuroneal differentiation [8] , [9] , [10] , [11] , we hypothesized that retrograde signals following axonal injury could lead to an epigenetic environmental shift facilitating the expression of genes critical to regeneration. We believed that a positive retrograde signal initiated by PNS injury could relax the chromatin environment surrounding specific promoters and allow for gene expression; however, a negative signal following CNS injury may restrict promoter accessibility and inhibit gene expression. Following equidistant CNS (dorsal column axotomy, DCA) or PNS (sciatic nerve axotomy, SNA) axotomies, from L4-L6 DRG we assessed both high-throughput promoter and CGI DNA methylation (DNA methylation microarrays) and histone modifications (quantitative chromatin immunoprecipitation (ChIP) assays) at the proximal promoters of genes previously established to be critical to regeneration such as growth-associated protein 43 (GAP-43) [12] , Galanin [13] and brain-derived neurotropic factor (BDNF) [14] , [15] ( Fig. 1a ). 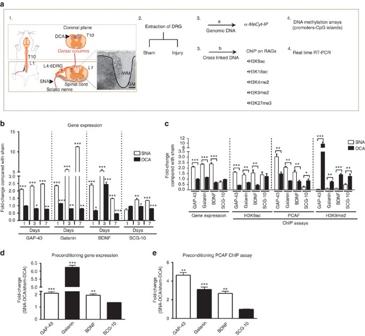Figure 1: H3K9ac and PCAF involvement in the regulation of regeneration genes. (a) Schematic diagram of SNA and DCA injury models used for epigenetic screens involving DNA methylation arrays and quantitative ChIP assays from L4-L6 DRG. Scale bar, 100 μm. (b) Fold change increases observed inGAP-43, GalaninandBDNFgene expression at 1, 3 and 7 days post SNA but not DCA and at 3 and 7 days forSCG-10. (c) Increased gene expression, H3K9ac, PCAF and decreased H3K9Me2 at GAP-43, Galanin and BDNF, but not SCG-10 (SCG-10 had decreased H3K9me2 enrichment to a lesser extent) promoters following 1 day post-SNA versus DCA. (d) A preconditioning lesion performed 1 week before DCA still induced 24 h later gene expression ofGAP-43, GalaninandBDNFbut notSCG-10. (e) This correlated with an increase in PCAF at the promoters of activated regeneration genes. Q-PCR. (b,c)N=3 per group; ChIP assays (c–e)N=6 per group, Student’st-test, error bars, s.e. *P<0.05, **P<0.01, ***P<0.001. All experiments were performed in triplicate. Figure 1: H3K9ac and PCAF involvement in the regulation of regeneration genes. ( a ) Schematic diagram of SNA and DCA injury models used for epigenetic screens involving DNA methylation arrays and quantitative ChIP assays from L4-L6 DRG. Scale bar, 100 μm. ( b ) Fold change increases observed in GAP-43, Galanin and BDNF gene expression at 1, 3 and 7 days post SNA but not DCA and at 3 and 7 days for SCG-10 . ( c ) Increased gene expression, H3K9ac, PCAF and decreased H3K9Me2 at GAP-43, Galanin and BDNF, but not SCG-10 (SCG-10 had decreased H3K9me2 enrichment to a lesser extent) promoters following 1 day post-SNA versus DCA. ( d ) A preconditioning lesion performed 1 week before DCA still induced 24 h later gene expression of GAP-43, Galanin and BDNF but not SCG-10 . ( e ) This correlated with an increase in PCAF at the promoters of activated regeneration genes. Q-PCR. ( b , c ) N =3 per group; ChIP assays ( c – e ) N =6 per group, Student’s t -test, error bars, s.e. * P< 0.05, ** P< 0.01, *** P< 0.001. All experiments were performed in triplicate. Full size image DNA methylation arrays showed a modest number of genes differentially methylated between injuries ( Supplementary Fig. 1a–e ); however, none of the genes associated with regeneration displayed significant levels of methylation nor were they differentially methylated between SNA and DCA ( Supplementary Fig. 2a ). More importantly, and as opposed to a recent study investigating folate and its DNA methylation after sciatic and spinal injury [16] , quantitative RT–PCR analysis of the differentially methylated genes, and DNA methyltransferases did not show a consistent correlation between DNA methylation levels and gene expression ( Supplementary Figs 2b–e and 3 ). Therefore, promoter and CGI DNA methylation does not appear to be a key factor in the differential regenerative response between CNS and PNS injuries in the DRG system. Next, we investigated whether key histone modifications would be specifically enriched on established critical genes for the regenerative programme in DRG neurones. Of all histone modifications that correlate with active gene transcription (H3K9ac, H3K18ac, H3K4me2) [17] or gene repression (H3K9me2 and H3K27me3) [17] that were screened, H3K9ac, H3K9me2 and H3K27me3 were enriched compared with IgG on most promoters; however, only H3K9ac and H3K9me2 were found to be differentially enriched at GAP-43 , Galanin and BDNF promoters, consistently correlating with early and sustained increased expression following SNA (1–7 days; Figs 1b,c and 2a–d ; Tables 1 and 2 ). Additionally, these three genes presented common promoter motifs in CpG content as well as transcription-binding sites that together with increased H3K9ac at their promoters suggest common transcriptional regulation ( Fig. 1b,c ). H3K9ac and the H3K9ac-specific acetyltransferase, PCAF, are typically found in the proximity of transcriptional start sites of actively transcribing genes [17] , and accordingly PCAF was also enriched at these promoters ( Fig. 1c ). Interestingly, H3K9me2, which is associated with gene silencing [17] , was found to be decreased at these promoters and inversely correlated to gene expression following SNA ( Fig. 1c ). In contrast, SCG-10 , whose gene expression is unaltered after 24 h and only modestly increased following 3- and 7-day SNA ( Fig. 1b ), did not show an enhancement of H3K9ac or PCAF at its promoter ( Fig. 1c ). Given that a preconditioning lesion (SNA preceding DCA) activates the regenerative capacity of the CNS [7] , we questioned whether a PNS epigenetic signal overrides a CNS signal. We observed an increase in the gene expression of these genes following preconditioned DCA versus DCA alone, which correlated with an increase in PCAF at these promoters ( Fig. 1d,e ). Furthermore, a broader picture of post-axotomy gene expression profiles and H3K9ac promoter enrichment is depicted by regeneration-associated ( Chl1, L1cam, SPRR1a ) [18] , axonal growth ( ATF3 and Bcl-xL ) [19] , [20] housekeeping ( ribosomal unit 18S ) genes and axonal structure ( NF-L ) genes [21] ( Fig. 2a,b ). Importantly, these experiments show that H3K9ac, a marker of actively transcribing genes, is selectively enriched on the promoters of GAP-43 , Galanin and BDNF , but not on the promoters of other SNA-induced genes such as SPRR1a , ATF3 and HSP27 ( Fig. 2a–d ; Table 1 ), suggesting that their common regulation maybe linked to their importance in regeneration. 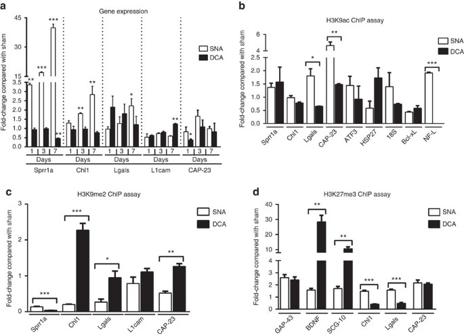Figure 2: Histone modifications that do not correlate with gene expression. (a) Gene expression of genes associated with regeneration found to be induced (Sprr1aandChl1) or not changed (Lgals, L1camandCAP-23) at various timepoints. (b) H3K9ac ChIP assays at the promoters of several genes previously found to be either induced (Sprr1a,HSP27andATF3), unchanged (Chl1and18S) or repressed (Bcl-xLandNF-L) in gene expression 24 h post SNA only showed a correlation between expression and H3K9ac promoter occupancy for Bcl-xL. No enrichment to IgG was found for L1cam promoter. (c) ChIP assay for H3K9me2 24 h post SNA and DCA compared with Shams shows no correlation with 24-h gene expression time point for Sprr1a, Chl1, Lgals and CAP-23, but for L1cam there is no change observed, which is in agreement with no change in gene expression. (d) No consistent pattern of correlation with gene expression was found with H3K27me3 24 h post SNA by ChIP assay. No enrichment was found compared with IgG for L1cam and Galanin. (ChIP assays,N=6 per group, performed in triplicate). Error bars, s.e. (a,c,d) Student’st-test, *P<0.05, **P<0.001 and ***P<0.001. Figure 2: Histone modifications that do not correlate with gene expression. ( a ) Gene expression of genes associated with regeneration found to be induced ( Sprr1a and Chl1 ) or not changed ( Lgals, L1cam and CAP-23 ) at various timepoints. ( b ) H3K9ac ChIP assays at the promoters of several genes previously found to be either induced ( Sprr1a , HSP27 and ATF3 ), unchanged ( Chl1 and 18S ) or repressed ( Bcl-xL and NF-L ) in gene expression 24 h post SNA only showed a correlation between expression and H3K9ac promoter occupancy for Bcl-xL. No enrichment to IgG was found for L1cam promoter. ( c ) ChIP assay for H3K9me2 24 h post SNA and DCA compared with Shams shows no correlation with 24-h gene expression time point for Sprr1a, Chl1, Lgals and CAP-23, but for L1cam there is no change observed, which is in agreement with no change in gene expression. ( d ) No consistent pattern of correlation with gene expression was found with H3K27me3 24 h post SNA by ChIP assay. No enrichment was found compared with IgG for L1cam and Galanin. (ChIP assays, N =6 per group, performed in triplicate). Error bars, s.e. ( a , c , d ) Student’s t -test, * P< 0.05, ** P< 0.001 and *** P< 0.001. Full size image Table 1 Correlation between gene expression and H3K9ac ChIP data. Full size table Table 2 Enrichment of histone modifications over IgG. Full size table NGF-MEK-ERK signalling regulates PCAF and H3K9ac Next, we turned our attention to understanding whether retrograde signalling following SNA plays a role in this positive chromatin remodelling. Immediately following peripheral injury, pERK levels rise in the injured axon and ERK signalling modules are retrogradely transported to the DRG cell body [22] , [23] , where we show that global PCAF and H3K9ac levels rise ( Fig. 3a–c ). In adult primary DRG neuroneal cultures, nerve growth factor (NGF), an activator of ERK signalling and neurite outgrowth [24] , increased the expression of PCAF and H3K9ac, while the ERK kinase (MEK) inhibitor, PD98059 (PD), prevented PCAF and H3K9ac induction [25] ( Fig. 4a,b ). NGF induces PCAF expression, nuclear localization and activation of acetyltransferase activity specifically by threonine phosphorylation at its histone acetyltransferase domain [26] . In L4-L6 DRG, SNA induced the expression of nuclear PCAF and PCAF threonine but not serine phosphorylation ( Fig. 4c,d ). This correlated with an increase in pERK in DRG, as well as nuclear PCAF translocation and acetylation of H3K9, all of which are dependent on ERK activation following SNA ( Fig. 4e–i ). As predicted, inhibition of ERK activation following SNA decreased gene expression as well as PCAF and H3K9ac at the promoters of GAP-43 , Galanin and BDNF ( Fig. 4j–l ). However, in conjunction with our theory of specificity of regulation, H3K9ac did not correlate with gene expression at other promoters following inhibition of ERK activation ( Supplementary Fig. 4a,b ). Remarkably, cAMP signalling in adult DRG neuroneal cultures did not induce nuclear PCAF translocation ( Supplementary Fig. 5 ), suggesting that cAMP-mediated mechanisms only partially supporting conditioning-dependent axonal regeneration [27] operate independently from pERK-induced epigenetic PCAF-mediated long-term mechanisms. These data present the first link between retrogradely transported PNS-injury-related signals and epigenetic modifications at the promoters of specific established regenerative genes. 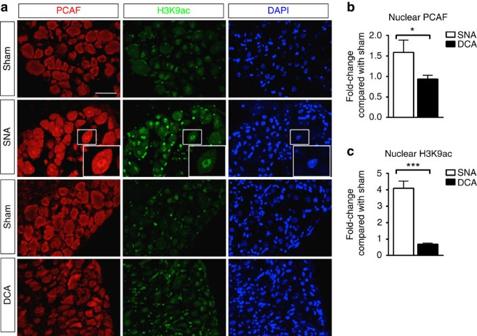Figure 3: Increased nuclear PCAF and H3K9ac following SNA but not DCA. (a) IHC co-staining with PCAF and H3K9ac of L4-L6 DRG following Sham/SNA or Sham/DCA. Insert shows high nuclear expression of PCAF and H3K9ac after SNA. Scale bar, 50 μm. (b) IHC intensity density analysis reveals an increase in nuclear PCAF following SNA/Sham but not DCA/Sham. (c) Intensity density analysis of IHC stained with H3K9ac reveals a significant fold increase following SNA but not DCA when compared with respective Sham. Student’st-test, error bars, s.e., *P<0.05, ***P<0.001,N=3 per group, performed in triplicate. Figure 3: Increased nuclear PCAF and H3K9ac following SNA but not DCA. ( a ) IHC co-staining with PCAF and H3K9ac of L4-L6 DRG following Sham/SNA or Sham/DCA. Insert shows high nuclear expression of PCAF and H3K9ac after SNA. Scale bar, 50 μm. ( b ) IHC intensity density analysis reveals an increase in nuclear PCAF following SNA/Sham but not DCA/Sham. ( c ) Intensity density analysis of IHC stained with H3K9ac reveals a significant fold increase following SNA but not DCA when compared with respective Sham. Student’s t -test, error bars, s.e., * P< 0.05, *** P< 0.001, N =3 per group, performed in triplicate. 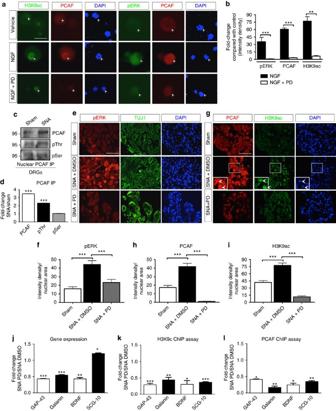Figure 4: ERK retrograde signalling controls PCAF activation. (a,b) NGF stimulates pERK, PCAF and H3K9ac expressions in adult DRG cultures after 3-h treatment, which is abrogated by the ERK kinase inhibitor PD98059 (PD), ICC (a) and fold change analysis of intensity density (b). Scale bar, 20 μm,N=3 per group, performed in triplicate. (c,d) Nuclear PCAF immunoprecipitation fromin vivoL4-L6 DRG 24 h following Sham or SNA reveals an increase in PCAF expression and threonine phosphorylation following SNA but not serine phosphorylation, immunoblot (c) and fold change of density analysis (d).N=5 per group, performed in triplicate. (e–i) In L4-L6 DRG, 24 h following SNA we observe an increase in pERK (e,f), PCAF (g,h) and H3K9ac (g,i) expression, which is significantly decreased by ERK inhibition with PD at the nerve stump. Insert shows high nuclear expression of PCAF and H3K9ac after SNA. Scale bars, 75 μm,N=3 per group, performed in triplicate. (j–l) PD also inhibits gene expression (Q-PCR,N=3 per group) (j) as well as H3K9ac (k) and PCAF (l) at the promoters of GAP-43, Galanin and BDNF 24 h following SNA (ChIPs).N=6 per group, performed in triplicate. Error bars, s.e. (b,f,h,i)P<0.0001, ANOVA, Bonferronipost hoctests, **P<0.001 and ***P<0.001, (d,j–l) Student’st-test, *P<0.05, **P<0.001 and ***P<0.001. Original immunoblot images are shown inSupplementary Fig. 12. Full size image Figure 4: ERK retrograde signalling controls PCAF activation. ( a , b ) NGF stimulates pERK, PCAF and H3K9ac expressions in adult DRG cultures after 3-h treatment, which is abrogated by the ERK kinase inhibitor PD98059 (PD), ICC ( a ) and fold change analysis of intensity density ( b ). Scale bar, 20 μm, N =3 per group, performed in triplicate. ( c , d ) Nuclear PCAF immunoprecipitation from in vivo L4-L6 DRG 24 h following Sham or SNA reveals an increase in PCAF expression and threonine phosphorylation following SNA but not serine phosphorylation, immunoblot ( c ) and fold change of density analysis ( d ). N =5 per group, performed in triplicate. ( e – i ) In L4-L6 DRG, 24 h following SNA we observe an increase in pERK ( e , f ), PCAF ( g , h ) and H3K9ac ( g , i ) expression, which is significantly decreased by ERK inhibition with PD at the nerve stump. Insert shows high nuclear expression of PCAF and H3K9ac after SNA. Scale bars, 75 μm, N =3 per group, performed in triplicate. ( j – l ) PD also inhibits gene expression (Q-PCR, N =3 per group) ( j ) as well as H3K9ac ( k ) and PCAF ( l ) at the promoters of GAP-43, Galanin and BDNF 24 h following SNA (ChIPs). N =6 per group, performed in triplicate. Error bars, s.e. ( b , f , h , i ) P< 0.0001, ANOVA, Bonferroni post hoc tests, ** P< 0.001 and *** P< 0.001, ( d , j – l ) Student’s t -test, * P< 0.05, ** P< 0.001 and *** P< 0.001. Original immunoblot images are shown in Supplementary Fig. 12 . Full size image PCAF supports axonal regeneration mimicking a conditioning lesion As a preconditioning lesion is able to induce neurite outgrowth in primary adult DRG neurones cultured on permissive (laminin) or non-permissive (myelin) substrates [28] , we tested whether increased PCAF expression by adeno-associated virus (AAV, Supplementary Fig. 6a–c ) could also drive neurite outgrowth. Indeed, neurite outgrowth increased on laminin and myelin by PCAF overexpression in DRG ( Fig. 5a,b ) as well as another CNS primary culture, cerebellar granule neurones (CGN, Supplementary Fig. 7a ). In CGN (employed for its ease of culture and greater cell number for use in immunobloting, ChIP and transfections for luciferase assays) there was a significant decrease in H3K9ac when plated on myelin ( Supplementary Fig. 7b,c ) and a reduction of H3K9ac at select promoters, which was reverted to permissive levels with overexpression of PCAF ( Supplementary Fig. 7d ). Likewise, PCAF overexpression reversed myelin repression of select genes in DRGs ( Fig. 5c ). Furthermore, the drug Garcinol (5 μM), which inhibits PCAF acetyltransferase activity [29] , reduced neurite outgrowth in DRG ( Fig. 5d,e ) and CGN ( Supplementary Fig. 7e,f ), decreased the luciferase expression of a GAP-43 promoter luciferase construct in CGN ( Supplementary Fig. 7g ) and decreased select gene expression in DRG ( Fig. 5f ). In ex vivo experiments, the inhibition of PCAF activity by Garcinol was able to significantly limit neurite outgrowth on both laminin and myelin as well as repress H3K9ac induced by SNA ( Fig. 5g–i ). Correspondingly, PCAF−/− mice provided full abolishment of neurite outgrowth induced by SNA in ex vivo cultured DRG neurones ( Fig. 5j,k ). Additionally, SNA-dependent neurite outgrowth in ex vivo cultured DRG neurones was blocked by ERK inhibition via delivery of PD at the nerve stump ( Fig. 6a–c ), phenocopying PCAF loss of function experiments. 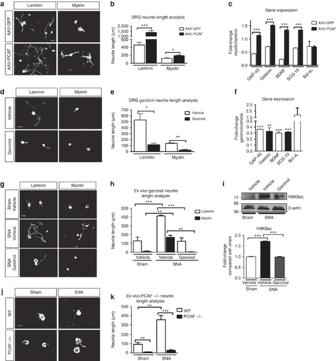Figure 5: PCAF promotes neurite outgrowthin vitroandex vivofollowing SNA. (a,b) On both laminin and myelin substrates, adult DRG infected with AAV-PCAF (48 h) showed an increase in neurite outgrowth compared with AAV-GFP-infected DRG, ICC (βIII Tubulin) (a) and average neurite length analysis (b). Scale bars, 100 μm. (c) Q-PCR fold changes of myelin/laminin 48-h post-AAV infection reveals inhibitory myelin-dependent reduction in gene expression of regeneration genes, which was restored by PCAF overexpression. (d–f) On laminin and myelin substrates, the PCAF activity inhibitor Garcinol (24 h) represses neurite outgrowth as well as the gene expression of regeneration genes, ICC (βIII Tubulin) Scale bars, 50 μm (d), average neurite length analysis (e) and Q-PCR (f–i) Garcinol when applied intrathecally compared with Vehicle at the time of a conditioning lesion significantly repressed neurite outgrowth of the given lesion 24 h later inex vivocultures on both laminin and myelin substrates as well as the acetylation of H3K9, ICC (βIII Tubulin). Scale bars, 50 μm (g), average neurite length analysis (h) and western blot and intensity analyses (i). (j,k) In addition, neurite outgrowth inex vivocultures from PCAF−/− mice showed PCAF to be required for neurite outgrowth induced by a conditioning lesion, ICC (βIII Tubulin). Scale bars, 50 μm (j), average neurite length analysis (k). Error bars, s.e. (b,c,e,h,i,k)P<0.0001, ANOVA, Bonferronipost hoctests, *P<0.05, **P<0.001 and ***P<0.001. (f) Student’st-test, **P<0.001 and ***P<0.001,N=3–6, performed in triplicate. Original immunoblot images are shown inSupplementary Fig. 13. Figure 5: PCAF promotes neurite outgrowth in vitro and ex vivo following SNA. ( a , b ) On both laminin and myelin substrates, adult DRG infected with AAV-PCAF (48 h) showed an increase in neurite outgrowth compared with AAV-GFP-infected DRG, ICC (βIII Tubulin) ( a ) and average neurite length analysis ( b ). Scale bars, 100 μm. ( c ) Q-PCR fold changes of myelin/laminin 48-h post-AAV infection reveals inhibitory myelin-dependent reduction in gene expression of regeneration genes, which was restored by PCAF overexpression. ( d – f ) On laminin and myelin substrates, the PCAF activity inhibitor Garcinol (24 h) represses neurite outgrowth as well as the gene expression of regeneration genes, ICC (βIII Tubulin) Scale bars, 50 μm ( d ), average neurite length analysis ( e ) and Q-PCR ( f – i ) Garcinol when applied intrathecally compared with Vehicle at the time of a conditioning lesion significantly repressed neurite outgrowth of the given lesion 24 h later in ex vivo cultures on both laminin and myelin substrates as well as the acetylation of H3K9, ICC (βIII Tubulin). Scale bars, 50 μm ( g ), average neurite length analysis ( h ) and western blot and intensity analyses ( i ). ( j , k ) In addition, neurite outgrowth in ex vivo cultures from PCAF−/− mice showed PCAF to be required for neurite outgrowth induced by a conditioning lesion, ICC (βIII Tubulin). Scale bars, 50 μm ( j ), average neurite length analysis ( k ). Error bars, s.e. ( b , c , e , h , i , k ) P< 0.0001, ANOVA, Bonferroni post hoc tests, * P< 0.05, ** P< 0.001 and *** P< 0.001. ( f ) Student’s t -test, ** P< 0.001 and *** P< 0.001, N =3–6, performed in triplicate. Original immunoblot images are shown in Supplementary Fig. 13 . 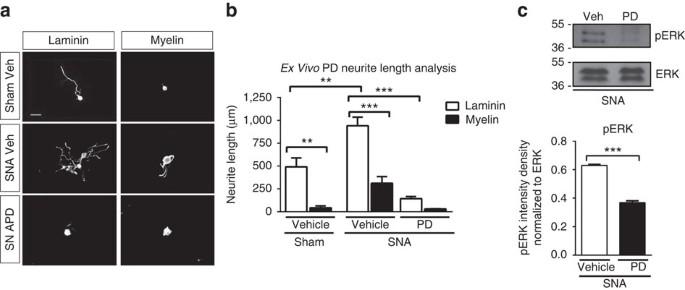Figure 6: ERK kinase inhibition blocks neurite outgrowth after conditioning lesion. (a–c) PD98059 when applied at the nerve stump compared with Vehicle at the time of a conditioning lesion or in Sham significantly repressed neurite outgrowth 12 h later inex vivocultures on both laminin and myelin substrates, ICC (βIII Tubulin). Scale bars, 50 μm (a), average neurite length analysis (b) and western blot and intensity analysis showing significant reduction in pERK after PD98059 delivery (c). (b)P<0.0001, ANOVA, Bonferroni post hoc tests, **P<0.001 and ***P<0.001. (c) Student'st-test, ***P<0.001, N=3–6, performed in triplicate. Original immunoblot images are shown inSupplementary Fig. 14. Full size image Figure 6: ERK kinase inhibition blocks neurite outgrowth after conditioning lesion. ( a – c ) PD98059 when applied at the nerve stump compared with Vehicle at the time of a conditioning lesion or in Sham significantly repressed neurite outgrowth 12 h later in ex vivo cultures on both laminin and myelin substrates, ICC (βIII Tubulin). Scale bars, 50 μm ( a ), average neurite length analysis ( b ) and western blot and intensity analysis showing significant reduction in pERK after PD98059 delivery ( c ). ( b ) P <0.0001, ANOVA, Bonferroni post hoc tests, ** P <0.001 and *** P <0.001. ( c ) Student's t -test, *** P <0.001, N=3–6, performed in triplicate. Original immunoblot images are shown in Supplementary Fig. 14 . Full size image Thus far our data suggest that PCAF is integral to the signalling involved following PNS injury leading to regeneration by altering the epigenetic landscape and stimulating intrinsic competence through crucial gene expression. To validate these observations in vivo , we studied regeneration of ascending sensory fibres following a preconditioning lesion (SNA 7 days before DCA) in the absence of PCAF and found that PCAF is required for regeneration induced by a conditioning lesion and for the expression of GAP-43, Galanin and BDNF in DRG ( Fig. 7a–g ). Importantly, axonal tracing in SCI experiments in a cohort of PCAF-/- mice and strain-matched controls showed that PCAF-/- mice did not display any abnormalities or overt phenotype in axonal tracing or regarding the lesion site ( Fig. 7a ). 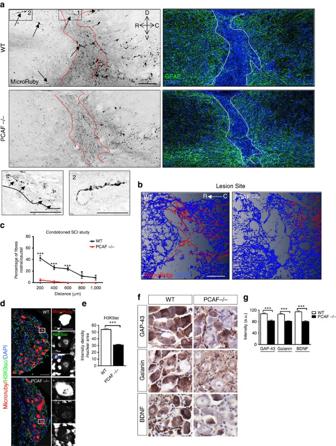Figure 7: PCAF is required for conditioning-dependent axonal regrowth after SCI. (a) MicroRuby tracing of the dorsal columns shows regenerating fibres invading into and past the lesion site (upper) in WT but not in PCAF−/− (lower) after conditioning injury (SNA followed by DCA; left panels). The red dotted lines indicate the lesion site. Insets (1 and 2) show higher magnification of regenerating axons. D-R-C-V: anatomical coordinates, dorsal-rostral-caudal-ventral. Right panels show the lesion site. Arrows indicate axonal sprouts. Scale bar, 100 μm. (b) Amira 3D reconstruction of regenerating dorsal column axons and glial scar in a sagittal projection (~25 μm) of the lesion site from WT and PCAF−/− mice. (c) Quantification of regenerating axons,N=6 (WT),N=6 (PCAF−/−), Welch’st-test, *P<0.05 and ***P<0.001. (d,e) Lack of CNS regeneration correlates with a significant decrease in H3K9ac expression in L4-L6 PCAF−/− traced DRG neurones when compared with WT, IHC (d), bar graphs (e). Inset shows high nuclear expression of H3K9ac in WT but not PCAF−/− traced DRG neurones. Student’st-test, error bars, s.e., ***P<0.001,N=6, performed in triplicate. (f,g) IHC and 3,3′-Diaminobenzidine (DAB) intensity analysis of L4-6 DRG neurones shows a decrease in GAP-43, BDNF and Galanin expression in PCAF−/− DRG neurones when compared with WT after SNA followed by SCI. Scale bar, 25 μm. Student’st-test, ***P<0.001,N=4 per group, performed in triplicate. Figure 7: PCAF is required for conditioning-dependent axonal regrowth after SCI. ( a ) MicroRuby tracing of the dorsal columns shows regenerating fibres invading into and past the lesion site (upper) in WT but not in PCAF−/− (lower) after conditioning injury (SNA followed by DCA; left panels). The red dotted lines indicate the lesion site. Insets (1 and 2) show higher magnification of regenerating axons. D-R-C-V: anatomical coordinates, dorsal-rostral-caudal-ventral. Right panels show the lesion site. Arrows indicate axonal sprouts. Scale bar, 100 μm. ( b ) Amira 3D reconstruction of regenerating dorsal column axons and glial scar in a sagittal projection (~25 μm) of the lesion site from WT and PCAF−/− mice. ( c ) Quantification of regenerating axons, N =6 (WT), N =6 (PCAF−/−), Welch’s t -test, * P< 0.05 and *** P< 0.001. ( d , e ) Lack of CNS regeneration correlates with a significant decrease in H3K9ac expression in L4-L6 PCAF−/− traced DRG neurones when compared with WT, IHC ( d ), bar graphs ( e ). Inset shows high nuclear expression of H3K9ac in WT but not PCAF−/− traced DRG neurones. Student’s t -test, error bars, s.e., *** P< 0.001, N =6, performed in triplicate. ( f , g ) IHC and 3,3′-Diaminobenzidine (DAB) intensity analysis of L4-6 DRG neurones shows a decrease in GAP-43, BDNF and Galanin expression in PCAF−/− DRG neurones when compared with WT after SNA followed by SCI. Scale bar, 25 μm. Student’s t -test, *** P< 0.001, N =4 per group, performed in triplicate. Full size image Next, we wondered whether PCAF overexpression alone would mimic regeneration induced by a conditioning lesion and enhance regeneration of ascending sensory fibres in the spinal cord following dorsal column lesion. Indeed, similar to that previously reported for a preconditioning lesion [7] , [30] , PCAF overexpression ( Supplementary Fig. 8 ) significantly increased the number of regenerating fibres across the lesion and up to a distance of 1 mm rostral of the lesion site ( Fig. 8a–c and Supplementary Fig. 9 ). Important to note, the depth of the lesion ( Supplementary Fig. 10 ) and lack of tracing rostral to the lesion site ( Supplementary Fig. 11 ) allowed excluding the presence of spared fibres. Furthermore, the introduction of the AAV directly into the sciatic nerve is in and of itself a PNS injury that does induce minimal sprouting towards the lesion in the GFP control. 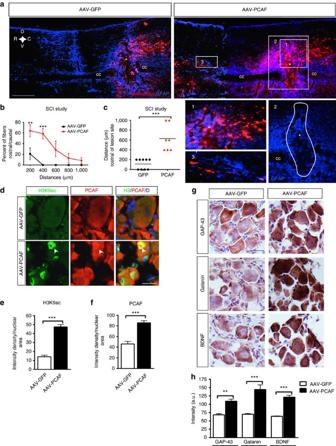Figure 8: PCAF overexpression induces spinal axonal regeneration. (a) MicroRuby tracing of the dorsal columns shows regenerating fibres invading into and past the lesion site after AAV-PCAF overexpression (upper right) versus a control AAV-GFP virus (upper left). Insets show higher magnification of regenerating axons. D-R-C-V: anatomical coordinates, dorsal-rostral-caudal-ventral. cc: central canal. Scale bar, 250 μm. (b) Quantification of regenerating axons,N=9 (AAV-GFP),N=7 (AAV-PCAF). (c) Quantification of longest regenerating axon per animal. (d–f) Overexpression of AAV-PCAF in the SCI study promotes H3K9ac (8 weeks post infection; arrowheads) as shown by IHC (d). Nuclear intensity density analysis of H3K9ac (e) and PCAF (f) show enhanced PCAF and H3K9ac after PCAF overexpression. (g,h) GAP-43, Galanin and BDNF IHC analysis of corresponding L4-L6 DRG from infected AAV-PCAF and AAV-GFP animals show an increase in GAP-43, Galanin and BDNF expression, IHC (g) and DAB intensity analysis (h). Scale bars, 25 μm. Error bars, s.e., (b) Welch’st-test, *P<0.05, **P<0.01 and ***P<0.001. (c,h)P<0.0001, ANOVA, Bonferronipost hoctests, **P<0.01 and ***P<0.001, (e,f) Student’st-test, ***P<0.001,N=3, performed in triplicate. Figure 8: PCAF overexpression induces spinal axonal regeneration. ( a ) MicroRuby tracing of the dorsal columns shows regenerating fibres invading into and past the lesion site after AAV-PCAF overexpression (upper right) versus a control AAV-GFP virus (upper left). Insets show higher magnification of regenerating axons. D-R-C-V: anatomical coordinates, dorsal-rostral-caudal-ventral. cc: central canal. Scale bar, 250 μm. ( b ) Quantification of regenerating axons, N =9 (AAV-GFP), N =7 (AAV-PCAF). ( c ) Quantification of longest regenerating axon per animal. ( d – f ) Overexpression of AAV-PCAF in the SCI study promotes H3K9ac (8 weeks post infection; arrowheads) as shown by IHC ( d ). Nuclear intensity density analysis of H3K9ac ( e ) and PCAF ( f ) show enhanced PCAF and H3K9ac after PCAF overexpression. ( g , h ) GAP-43, Galanin and BDNF IHC analysis of corresponding L4-L6 DRG from infected AAV-PCAF and AAV-GFP animals show an increase in GAP-43, Galanin and BDNF expression, IHC ( g ) and DAB intensity analysis ( h ). Scale bars, 25 μm. Error bars, s.e., ( b ) Welch’s t -test, * P< 0.05, ** P< 0.01 and *** P< 0.001. ( c , h ) P< 0.0001, ANOVA, Bonferroni post hoc tests, ** P< 0.01 and *** P< 0.001, ( e , f ) Student’s t -test, *** P< 0.001, N =3, performed in triplicate. Full size image Our work demonstrates that PCAF is required for conditioning-dependent spinal regeneration and that PCAF overexpression alone is able to promote regeneration of sensory fibres across the injured spinal cord and beyond similarly to previously established conditioning paradigms. Furthermore, PCAF-induced regeneration correlated with a significant increase in the expression of H3K9ac, GAP-43, Galanin and BDNF in the L4-L6 DRG. The definition of regeneration-associated genes (RAGs) is genes differentially induced between the regenerating PNS and non-regenerating CNS systems; however, this does not validate the entire class of genes as essential for immediate and sustained axonal regeneration. In support of this, our data show that PCAF-dependent regulation of GAP-43 , Galanin and BDNF is at the essential core of the regenerative programme. An immediate response to the external stimulus of a peripheral axonal injury is to seal the wound. This is followed by electrical impulses and calcium fluxes that are the first messages relayed from the lesion site to the cell body requesting assistance. Next, is a rise in cAMP levels and phosphorylation signalling by multiple players involved in transmitting further information to the cell body [5] , [6] . Recently, it has been shown that calcium influx ejects histone deacetylase 5 (HDAC5) from the DRG nucleus correlating to increased global H3ac and gene expression [31] . It has been hypothesized that merely shifting the balance from a deacetylated to a globally acetylated chromatin environment by inhibition of HDACs could recapitulate the conditioning lesion and could lead to regeneration. However, recent experimental evidence [32] and our own work using HDAC class I and HDAC class I and II inhibitors [33] has proven this to be insufficient in producing post-lesion regeneration of sensory fibres following a spinal or optic nerve injury and therefore unlikely the key to unlocking the molecular mechanisms of regeneration. While our work here describes that specific epigenetic codes are induced endogenously following a conditioning lesion that leads to CNS regeneration, it is also consistent with previous findings from our laboratory that showed the presence of a transcriptional complex formed by p53, p300 and PCAF in the proximity of several RAGs including GAP-43 , Coronin 1b and Rab13 in primary neurones as well as facial motor neurones in a PNS facial nerve axotomy model [34] , [35] , [36] . Additionally, we found that the histone acetyltransferase p300 (which may form a complex with PCAF) is developmentally regulated in retinal ganglion cells and whose overexpression drives axonal regeneration of the injured optic nerve [33] . While it is known that signals are sent via retrograde transport machinery [23] , [37] , [38] , [39] , how they are decoded into the gene expression of key axonal regeneration players for growth towards re-innervation of the lost target has not been known until now. Here, we have shown the first systematic study of various epigenetic modifications revealing specifically that increased H3K9ac and PCAF as well as decreased H3K9me2 at the promoters of GAP-43 , Galanin and BDNF are due to retrogradely induced pERK activation of PCAF leading to essential gene activation, which is sufficient to mimic the regenerative response assembled by a conditioning lesion, thus driving regeneration in the CNS. The fundamentals of decoding the regenerative retrograde signal by understanding the specific epigenetic changes that occur to chromatin surrounding essential genes is paramount in our ability to recapitulate this mechanism when the signal is lacking, such as after spinal cord injury (SCI). Here we take the first steps in this understanding that may lead to the design of epigenetic-related regenerative therapies for SCI patients. Reagents PD 98059 (Calbiochem), Garcinol (Sigma-Aldrich), NGF (BD Biosciences) and dbcAMP (Enzo Life Sciences) were purchased from respective companies. The following antibodies were purchased and utilized, rabbit anti-PCAF (ab12188, Abcam), mouse anti-PCAF (E8, sc-13124, Santa Cruz Biotechnology), rabbit anti-AcH3K9 (no. 9671, Cell Signalling), rabbit anti-H3K9me2 (no. 9753, Cell Signalling), mouse anti-H3K27me3 (ab6002, Abcam), mouse anti-H3K4me2 (no. 9726, Cell Signalling), rabbit anti-H3K18ac (ab15823, Abcam), mouse anti-NeuN (MAB 377, Millipore), rabbit anti-phospho-Erk 1/2 (no. 9101, Cell Signalling), mouse anti-ßIII tubulin (no. G712A, Promega), mouse β-actin (A2228, Sigma), rabbit anti-Phospho-Threonine (no. 600-403-263, Rockland), rabbit anti-Phospho-Serine (no. ADI-KAP-ST2103-E, Enzo Life Sciences), rabbit anti-MAP2 (sc20172, Santa Cruz Biotechnology), rat anti-Glial fibrillary acidic protein (GFAP) (no. 13-0300, Invitrogen), rabbit anti-BDNF (sc-546, Santa Cruz Biotechnology), rabbit anti-Galanin (T-4334, Bachem Peninsula Laboratories) and sheep anti-GAP-43 (no. NBP1-41123, Novus Biologicals). Mice All mice used for this work were treated according to the Animal Welfare Act and to the ethics committee guidelines of the University of Tu¨bingen. Equally distributed male and female C57Bl6/J (bred from Charles River Laboratories), CD1 or CD1 PCAF−/− (generated in Dr Boutillieŕs laboratory) mice ranging from 6 to 8 weeks of age were used for all experiments. C57Bl6/J were used for all studies except those specifying PCAF null mice. For surgeries, mice were anesthetized with ketamine (100 mg kg −1 body weight) and xylazine (10 mg kg −1 body weight). For all experiments, we employed a target for the appropriate expected power calculation linked to an ad hoc statistical test. Dorsal column axotomy Surgeries were performed as previously reported [40] . Briefly, mice were anesthetized and a T10 laminectomy was performed (~20 mm from the L4-L6 DRGs), the dura mater was removed, taking care of not damaging the spinal cord. A dorsal hemisection until the central canal was performed with a microknife (FST). For the control laminectomy surgery, the dura mater was removed but the dorsal hemisection was not performed. Sciatic nerve axotomy Mice were anesthetized. At ~20 mm far from L4-L6 DRG, a 10-mm incision was performed on the gluteal region and muscles were displaced to expose the sciatic nerve for a complete transection with spring micro-scissors. For the PD study 30 s before transection, 2.5 μl of 100% DMSO or 2.0 μl of PD 98059 were slowly pipetted on the nerve. Finally, skin was closed with two suture clips. The nerve fibre was left uninjured in sham surgery. Methylated DNA immunoprecipitation from DRG ex vivo For each of the three time points (1, 3 and 7 days post SNA or DCA and naive), L4-L6 DRG were collected from two mice per time point and condition in triplicate for injury samples and naive, and in duplicate for shams. Frozen tissue was ground and digested with 0.2 mg ml −1 Proteinase K. The lysate was then sonicated to average size of 700 bp and cleared of remaining tissue by centrifugation. Genomic DNA was extracted from the lysate via standard phenol–chloroform extraction and DNA precipitation protocols. MeDIP was then performed according to the manufacturer’s protocol for the ChIP Kit from Upstate/Millipore. A total of 10 μg of genomic DNA and 5 μg of a 5-methyl-Cytosine antibody (Eurogentec, BI-MECY-0100) were added to immunoprecipitate methylated DNA fragments. The Whole Genome Amplification Kit (Sigma-Aldrich) was applied to amplify 20 ng of genomic samples to a maximum yield of 3–7 μg, followed by subsequent column purification using the GenElute PCR Clean-Up Kit (Sigma). MeDIP efficiency was tested with previously published primers for methylated H19 ICR [41] . DNA methylation microarray Whole-genome amplified, high-quality [42] samples (input genomic DNA, immunoprecipitated methylated DNA or no-antibody control) were sent to Roche/NimbleGen for DNA methylation microarray analysis. NimbleGen processed the samples as described in its ‘NimbleChip Arrays User’s Guide for DNA Methylation Analysis’. A ‘2007-02-27 MM8 CpG Island Promoter (385K RefSeq)’ tiling microarray, covering proximal promoter regions and CGIs by close-set oligonucleotide probes. Fluorescence intensity raw data were obtained from scanned images of the tiling arrays using the NimbleScan extraction software. For each spot on the array, Cy5/Cy3 ratios were normalized and calculated to obtain log2 values. Then, the bi-weight mean of log2 ratios of a certain region was subtracted from each data point; this procedure is similar to mean normalization of each channel. Promoter CGI analysis Several known RAGs and of differentially methylated genes that emerged from the DNA methylation microarray analysis within this study were analyzed for CpG islands (CGIs). The complete genomic region, together with the promoter region (5,000 bp upstream of the transcription start site (TSS)), was analysed with the EMBOSS CpGPlot online tool from EMBL-EBI. Characteristic parameters of reported CGIs were used. Gene-regulatory region bioinformatics analysis We performed a Matinspector (Genomatix) and UCSD genome browser-based bioinformatics analysis of the regulatory regions of RAG genes ( GAP-43 , Galanin , BDNF , SCG-10 , Sprr1a , Chl1 , Lgals , L1cam and CAP-23 ) spanning 1,000 bp upstream and 1,500 bp downstream of the TSS. These regions overlap and further extend what we studied for DNA methylation (500 bp upstream and 1,500 bp downstream of the TSS). Significant transcription-binding sites displayed at least two of the three classically required criteria: a P- value <0.05, matrix similarity >0.8 and core similarity >0.8. Additionally, CGI and DNA methylation were examined in these regions for all of the RAGs investigated with the EMBO DNA methylation analysis online software. Results of the combined analysis suggested that GAP-43, Galanin and BDNF had common gene regulatory regions with low levels of DNA methylation and absence of typical CpG islands, presented transcriptional-binding sites for transcription factors that are typically acetylated and active in the proximity of acetylated histones, including, Klf, NFkB, SRF, p53, YY1, CREB and c-jun. Quantitative real-time RT–PCR analysis RNA was extracted using PeqGOLD TriFast reagent (peqlab), cDNA was synthesized from 1 μg of total RNA using both oligodT and random hexamers from the SuperScript II Reverse Transcriptase kit (Invitrogen) and a real time RT–PCR was performed using Absolute QPCR SYBR low ROX master mix (Thermo Scientific). Quantities and fold changes were calculated following the manufacturer’s instructions (ABI 7,500) and as previously reported [35] , [43] . Primer sequences are shown in Supplementary Table 1 . RPL13A, GAPDH or β-actin were used for normalization. Quantitative chromatin immunoprecipitation The SimpleCHIP Enzymatic Chromatin IP Kit with magnetic beads (Cell Signalling) was used according to previously published methods [44] . Antibodies used were H3K9ac, PCAF (rabbit), H3K9me2, H3K27me3, H3K4me3 and H3K18ac. Real-time Q-PCR was run using Absolute QPCR SYBR low ROX master mix (Thermo Scientific). Quantities and fold changes were calculated following the manufacturer’s instructions (ABI 7,500) and as previously reported [35] , [43] . Primers were designed in proximity (within 500 bp upstream) of the TSS. Primer sequences are shown in Supplementary Table 2 . Immunohistochemistry DRG were fixed in 4% paraformaldehyde (PFA) and transferred to 30% sucrose. The tissue was embeded in OCT compound (Tissue-Tek), frozen at −80 °C and sectioned at 10-μm thickness. DRG sections underwent antigen retrieval with 0.1 M citrate buffer (pH 6.2) at 98 °C and were incubated with 120 μg ml −1 goat anti-mouse IgG (Jackson Immunoresearch). They were blocked for 1 h with 8% BSA, 1% PBS-TX100 or 0.3% PBS-TX100, respectively, and then incubated with NeuN (1:100), PCAF (mouse, 1:500) and AcH3K9 (1:500) antibodies or phospho-Erk 1/2 (1:500) and ßIII tubulin (1:1,000) antibodies O/N. This was followed by incubation with Alexa Fluor 568-conjugated goat anti-mouse and Alexa Fluor 488-conjugated goat anti-rabbit or Alexa Fluor 568-conjugated goat anti-rabbit and Alexa Fluor 488-conjugated goat anti-mouse (1:1,000, Invitrogen), respectively. Slides were counterstained with DAPI (1:5,000, Molecular Probes). Photomicrographs were taken with an Axio Imager.Z1/Apotome (Zeiss) microscope as 0.800 μm Z-stacks at × 40 magnification and processed with the software AxioVision (Zeiss). In order to determine the nuclear intensity density (ID) of pixels, Image J (Fiji) was used. Each neuroneal nuclear area was selected in the DAPI channel (about 25 nuclei/picture). The same selection was then used to delineate the nuclei in the other channels. The threshold of the nuclear area was set for each different channels, and based on that the pixel ID of the nucleus was determined and divided by its nuclear area. Triplicates of each treatment were analysed. Immunoblotting and immunoprecipitation For whole-cell extract immunoblotting, DRG or CGN were collected, lysed on ice in RIPA lysis buffer containing protease inhibitors (Complete Mini; Roche Diagnostics), sonicated briefly, centrifuged and the supernatant collected. The NE-PER Nuclear and Cytoplasmic Extraction Reagents (Thermo Scientific) was used according to the manufacturer’s instructions for nuclear enriched fractions. H3K9ac (1:1,000), PCAF (rabbit,1:500), β-actin (1:1,000) and βIII Tubulin (1:1,000) were employed as primary antibodies. Quantitation of protein expression was performed by densitometry (Image J) of the representative bands of the immunoblots and normalized to the respective levels of loading controls. For immunoprecipitation, the nuclear enriched fractions were bound to rabbit PCAF antibody (8 μg), pulled down with Protein G magnetic beads, washed with low and high salt buffers (ChIP kit, Cell Signalling) and was eluted with loading buffer (Thermo Scientific). The IP was stained with PCAF (rabbit, 1:500), Phospho-Threonine (1:1,000) or Phospho-Serine (1:1,000). DRG culture Adult DRG were dissected and collected in Hank’s balanced salt solution on ice. DRGs were transferred to a digestion solution (5 mg ml −1 Dispase II (Sigma), 2.5 mg ml −1 Collagenase Type II (Worthington) in DMEM (Invitrogen)) and incubated at 37 °C for 35 min with occasional mixing. Following which DRGs were transferred to media containing 10% heat-inactivated fetal bovine serum (Invitrogen), 1 × B27 (Invitrogen) in DMEM:F12 (Invitrogen) mix and were briefly triturated with a Sigma-cote (Sigma) fire-polished pipette to manually dissociate the remaining clumps of DRG. After which the single cells were spun down, resuspended in media containing 1 × B27 and Penicillin/Streptomycin in DMEM:F12 mix and plated at 4,000–5,000 per coverslip. The culture was maintained in a humidified atmosphere of 5% CO 2 in air at 37 °C. Neurones were infected with either AAV-GFP or AAV-PCAF (1 × 10e12 ml −1 ) a few hours post-plating and fixed with 4% PFA 48 h later. For the Garcinol study, cells were exposed to Vehicle (5% EtOH) or Garcinol (5 μM per well, Sigma-Aldrich) for 24 h and fixed. For the ERK/PD study, the day following plating DRG were exposed for 1 h to PD 98059 (50 μM per well), then to NGF (100 ng ml −1 ) for 3 h and fixed. CGN culture CGNs were prepared from the cerebellum of 7-day-old C57Bl6/J mice following standard procedures [45] . These disassociated CGNs were plated on either PDL (with or without 5 μM Garcinol) or myelin for 24 h in a humidified atmosphere of 5% CO 2 in air at 37 °C. Neurones were infected at the time of plating with a CMV promoter AV-GFP or AV-PCAF (1 × 10e10 ml −1 ). Immunocytochemistry Glass coverslips were coated with 0.1 mg ml −1 PDL, washed and coated with mouse Laminin (2 μg ml −1 ; Millipore). For myelin experiments, they were additionally coated with 4 μg cm −2 rat myelin. Cells were plated on coated coverslips for 24 or 48 h, at which time they were fixed with 4% PFA/4% sucrose. Immunocytochemistry was performed as previously reported [45] using βIII Tubulin (1:1,000), MAP2 (1:100), PCAF (mouse, 1:400), AcH3K9 (1:1,000) or pErk1/2 (1:500). This was followed by incubation with Alexa Fluor 568-conjugated goat anti-mouse and Alexa Fluor 488-conjugated goat anti-rabbit (1:1,000, Invitrogen). To visualize the nucleus, we stained the cells with DAPI (1:5,000, Molecular Probes). Image analysis for immunocytochemistry DRG pictures were taken at × 20 magnification with an Axioplan 2 (Zeiss) microscope and processed with the software AxioVision (Zeiss). Using Image J, a threshold was set. On the basis of the threshold, for each picture the ID of pixels was calculated in each channel and then divided by its respective number of cells (about 225 cells per picture). This was carried out in triplicate. Neurite length analysis Immunofluorescence was detected using an Axiovert 200 microscope (Zeiss) and pictures were taken as a mosaic at × 10 magnification using a CDD camera (Axiocam MRm, Zeiss). Neurite analysis and measurements were performed using the Neurolucida software (MicroBrightField) in triplicate with 50 cells per triplicate. Luciferase assays Experiments were performed in CGN using electroporation with the rat neurone nucleofactor kit (Amaxa Biosystems) according to the provided protocol. Briefly, five million neurones were used for each cuvette, with 2–4 μg of total DNA (GAP-43-Luc reporter [46] and 25 ng of pRL-TK- Renilla -luciferase (Promega)). Neurones were plated in 24-well plates at a density of 0.4 million cells per well with or without 5 μM Garcinol and incubated for a total of 24 h. Cells were harvested and lysed with 100 μl of passive lysis buffer, and luciferase activities were determined using the Dual-Luciferase kit (Promega). Ex vivo DRG culture Intrathecal (i.t.) injection was performed using the Wilcox technique [47] . Mice were briefly anaesthesized with isofluorane (2%), and a lumbar cutaneous incision (1 cm) was made. I.t. injections were performed with 30-gauge 15-mm needles mated to a 5-μl luer tip syringe (Hamilton, Reno, NV, USA). The needle was inserted into the tissue between the L5 and L6 spinous processes and inserted ~0.5 cm with an angle of 20°. Vehicle (10% DMSO in 0.9% NaCl) or Garcinol (80 μM) was slowly injected in a final volume of 5 μl. Directly after i.t. injection of Vehicle or Garcinol, mice underwent Sham or SNA surgeries. Twenty-four hours after surgery, mice were killed and L4–L6 DRG were collected and cultured for 24 h, and were then fixed and stained. We used three animals per group and plated in triplicate. L4–L6 DRG were also collected for total protein extraction for western blot analysis of H3K9ac. For PCAF null ex vivo study, WT or PCAF−/− mice (generated in Dr Boutillier’s laboratory) underwent Sham or SNA surgeries. Twenty-four hours after surgery, mice were killed and L4–L6 DRG were collected and cultured for 18 h, and were then fixed and stained. We used three animals per group and the DRG were plated in triplicate. SCI study AAV-GFP/PCAF injection All experimental procedures were performed in accordance with protocols approved by the Univeristy of Tu¨bingen. PCAF expression plasmid was obtained from Addgene (Plasmid 8941). AAVs were prepared as described previously [48] . Mice were anaesthetized and the left sciatic nerve was injected with 1.5–2 μl of either AAV-GFP or AAV-PCAF (1 × 10e12 ml −1 ) using a glass-pulled micropipette. Standardized randomization and blinding strategies were adopted. Randomization of samples was performed by random assignment and labelling of control and test groups while between one to three experimenters were blind to the groups for each experiment performed. Spinal cord injury Two weeks after AAV injection, a T9–10 laminectomy was performed and the dorsal half of the spinal cord was crushed with no. 5 forceps (Dumont, Fine Science Tools) for 2 s (ref. 49 ). The forceps were deliberately positioned to severe the dorsal column axons completely. Four weeks after the spinal cord lesion, dorsal column axons were traced by injecting 2 μl of Microruby tracer (3,000 molecular weight, 10%, Invitrogen) into the left sciatic nerve [50] . Mice were kept for an additional 2 weeks before termination. CD1 WT and PCAF−/− mice underwent the same spinal cord surgery as above. Additionally, they received a conditioning sciatic nerve lesion 1 week before the spinal surgery. One week after the spinal cord lesion, dorsal column axons were traced by injecting 2 μl of Microruby tracer (3,000 molecular weight, 10%, Invitrogen) into the left sciatic nerve [50] . These mice were kept for an additional 2 weeks before termination. Animals were deeply anaesthetized and were perfused transcardially. Spinal cords were dissected and post-fixed in 4% PFA in phosphate-buffered saline (PBS) at 4 °C for 2 h and 30% sucrose O/N. Then the tissue was embedded in Tissue-Tek OCT compound, frozen at −80 °C and cut in 18-μm-sagittal and coronal sections (3 mm caudal and 5 mm rostral to the lesion were taken to confirm the completeness of the lesion and to quantify tracing efficiency among experimental groups). Brain stem from each cord was also dissected, and sections of the nuclei gracilis and cuneatus were generated to monitor tracing from spared fibres. Mice with incomplete lesions were excluded. Staining for GFAP (1:2,000) was performed following the standard protocols [40] . Confocal laser scanning microscopy was performed using a Zeiss LSM700. Semi-automatic skeletonization of regenerating axons was performed on confocal scans using the three-dimensional (3D) imaging software Amira (FEI Visualization Sciences Group). An isosurface was applied to the GFAP signal. Quantification of axonal regeneration For each spinal cord after dorsal column crush, the number of fibres caudal to the lesion and their distance from the lesion epicentre were analysed in four to six sections per animal with a fluorescence Axioplan 2 (Zeiss) microscope and with the software StereoInvestigator 7 (MBF bioscience). The lesion epicentre (GFAP) was identified in each section at a × 40 magnification. The sum total number of labelled axons rostral to the lesion site was normalized to the total number of labelled axons caudal to the lesion site counted in all the analysed sections for each animal, obtaining an inter-animal comparable ratio considering the individual tracing variability. Sprouts and regrowing fibres were defined following the anatomical criteria reported by Steward et al. [51] Samples falling short of standard quality for each specific experiment or altered by clear experimental flaw were excluded from the analysis. DAB immunostaining Peroxidase activity was blocked in 0.3% H 2 O 2 , followed by incubation in 8% bovine serum albumin (BSA) and 0.3% TBS-TX-100. BDNF (1:500), Galanin (1:2,000) or GAP-43 (1:500) antibodies in 2% BSA and 0.2% TBS-TX100 were used. Labelled cells were visualized using the ABC system (Vectastain Elite; Vector Laboratories) with DAB as chromogen. The sections then were counterstained with haematoxylin (Vector Laboratories). Statistical analysis Data are plotted as the mean±s.e. All experiments were performed in triplicate. Asterisks indicate a significant difference analysed using analysis of variance with Bonferroni post hoc tests, Student’s t -test, Welch’s t -test or two-way analysis of variance as indicated (* P <0.05; ** P <0.01; *** P <0.001). Accession code: DNA methylation microarray data have been deposited in the NCBI Gene Expression Omnibus (GEO) database under the accession number GSE55514 . How to cite this article: Puttagunta, R. et al. PCAF-dependent epigenetic changes promote axonal regeneration in the central nervous system. Nat. Commun. 5:3527 doi: 10.1038/ncomms4527 (2014).